STIM1 triggers a gating rearrangement at the extracellular mouth of the ORAI1 channel The ER-resident regulatory protein STIM1 triggers store-operated Ca 2+ entry by direct interaction with the plasma membrane Ca 2+ channel ORAI1. The mechanism of channel gating remains undefined. Here we establish that STIM1 gates the purified recombinant ORAI1 channel in vitro , and use Tb 3+ luminescence and, separately, disulfide crosslinking to probe movements of the pore-lining helices. We show that interaction of STIM1 with the cytoplasmic face of the human ORAI1 channel elicits a conformational change near the external entrance to the pore, detectable at the pore Ca 2+ -binding residue E106 and the adjacent pore-lining residue V102. We demonstrate that a short nonpolar segment of the pore including V102 forms a barrier to ion flux in the closed channel, implicating the STIM1-dependent movement in channel gating. Our data explain the close coupling between ORAI1 channel gating and ion selectivity, and open a new avenue to dissect the gating, modulation and inactivation of ORAI-family channels. ORAI-family channels contribute to physiological Ca 2+ signalling in T cells and mast cells, and in skin, muscle and other tissues [1] , [2] , [3] , [4] . They have been implicated in pathological processes including immune disease, atherosclerosis and cancer progression [1] , [5] , [6] . The CRAC channel ORAI1 has served as the principal exemplar of ORAI-family channels, and its defining electrophysiological properties and the cellular processes leading to its activation have been well described [3] , [7] , [8] , [9] , [10] , [11] . However, electrophysiological investigation of ORAI channel gating is hindered by the slow process of activation in cells, in which STIM proteins must relocalize within the ER to ER-plasma membrane junctions [12] , [13] , [14] , and by the inability to resolve the very small currents through single ORAI channels [15] , [16] , [17] , [18] , [19] . Here we have investigated STIM-dependent gating with purified recombinant STIM1 cytoplasmic domain and purified recombinant ORAI1 channels. We have used the luminescence of Tb 3+ bound in the pore to probe conformational changes at the pore Ca 2+ -binding residue E106 in the wild-type human ORAI1 channel, and disulfide crosslinking to probe reorientation of the adjacent pore-lining residue 102 in an engineered V102C channel. The first main conclusion from these experiments is that STIM-dependent gating of the channel entails a structural change in the vicinity of residues E106 and V102 near the external entrance to the ORAI1 pore. Thus the close coupling of ORAI channel gating and ion selectivity reported in earlier studies [20] , [21] can be explained by STIM-dependent changes in ORAI pore architecture in a region critical for ion selectivity. The second main conclusion, from whole-cell recording of currents carried by engineered ORAI1 channels, is that a short nonpolar segment of the pore including V102 constitutes a barrier to ion flux in the closed ORAI channel. The structural rearrangement observed in this region of the pore is thus likely to be necessary for ion permeation. Overall, our study affords important new insight into STIM–ORAI signalling by directly probing STIM-dependent structural changes in the ORAI1 channel. Purified STIM1 and ORAI1 can reconstitute channel function The demonstration that purified STIM1 triggers Ca 2+ flux through purified recombinant ORAI channels is an essential prelude to biochemical studies of STIM–ORAI gating. We expressed human ORAI1 in Saccharomyces cerevisiae , purified the channel complex, and reconstituted it into liposomes ( Fig. 1a ). The liposomes contained Ca 2+ , whereas the surrounding solution was nominally Ca 2+ -free and contained the fluorescent Ca 2+ indicator Fura-2 ( Fig. 1b ). Addition of recombinant STIM1 cytoplasmic domain (STIM1 CT ) to the liposome suspension at concentrations from 20–100 μM caused an efflux of Ca 2+ from the liposomes that was detected as a shift in the excitation spectrum of Fura-2 ( Fig. 1c ). There was no efflux of Ca 2+ from negative control lipsomes reconstituted with the nonfunctional R91W ORAI1 channel [22] , [23] or from liposomes lacking the protein ( Fig. 1d,e ). The observations establish that recombinant STIM1 gates recombinant ORAI1 channels under the conditions used. 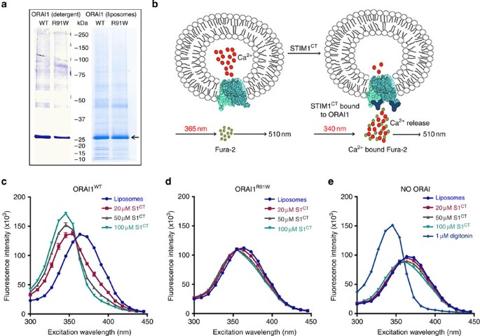Figure 1: STIM1 triggers Ca2+flux through reconstituted ORAI1 channels. (a) SDS–PAGE analysis of ORAI1WTand ORAI1R91Wproteins (marked by arrow) purified in the presence of decyl maltoside (two left lanes) and the same protein preparations after reconstitution into liposomes (two right lanes). (b) Ca2+flux assay to detect STIM1CT(S1CT)-mediated Ca2+release from liposomes through reconstituted ORAI1 channels (represented as cyan surface). Liposomes are generated with 5 mM Ca2+(red circles) inside. Free Fura-2 dye (green circles) devoid of Ca2+has an excitation peak at ~365 nm. Productive binding of STIM1CTto the ORAI1 channel causes Ca2+release from the liposomes, leading to a shift in the Fura-2 excitation peak to ~340 nm. Comparison of Fura-2 excitation scans of (c) liposomes containing ORAI1WT, (d) liposomes containing ORAI1R91Wand (e) liposomes without ORAI1 shows STIM1CT-mediated Ca2+release from ORAI1WTliposomes only. Digitonin was added at the end of each titration to establish that the liposomes contained releasable Ca2+, but this control is shown only for liposomes without ORAI protein. The liposome samples analysed inawere used for the experiments inc,d. Representative of three experiments. Figure 1: STIM1 triggers Ca 2+ flux through reconstituted ORAI1 channels. ( a ) SDS–PAGE analysis of ORAI1 WT and ORAI1 R91W proteins (marked by arrow) purified in the presence of decyl maltoside (two left lanes) and the same protein preparations after reconstitution into liposomes (two right lanes). ( b ) Ca 2+ flux assay to detect STIM1 CT (S1 CT )-mediated Ca 2+ release from liposomes through reconstituted ORAI1 channels (represented as cyan surface). Liposomes are generated with 5 mM Ca 2+ (red circles) inside. Free Fura-2 dye (green circles) devoid of Ca 2+ has an excitation peak at ~365 nm. Productive binding of STIM1 CT to the ORAI1 channel causes Ca 2+ release from the liposomes, leading to a shift in the Fura-2 excitation peak to ~340 nm. Comparison of Fura-2 excitation scans of ( c ) liposomes containing ORAI1 WT , ( d ) liposomes containing ORAI1 R91W and ( e ) liposomes without ORAI1 shows STIM1 CT -mediated Ca 2+ release from ORAI1 WT liposomes only. Digitonin was added at the end of each titration to establish that the liposomes contained releasable Ca 2+ , but this control is shown only for liposomes without ORAI protein. The liposome samples analysed in a were used for the experiments in c , d . Representative of three experiments. Full size image STIM1 elicits a conformational change near pore residue E106 A key part of our strategy was to observe conformational changes in the wild-type ORAI1 channel. Tb 3+ can serve as a luminescent probe of Ca 2+ binding sites in proteins. Tb 3+ binds to purified wild-type ORAI1 channels reconstituted into liposomes, as reported by enhanced Tb 3+ luminescence upon excitation at 280 nm ( Fig. 2a ). In line with the expectation that luminescence of Tb 3+ bound to protein is excited via aromatic side chains, the signal can be traced largely, but not exclusively, to energy transfer from residue Y115 in ORAI1 ( Supplementary Fig. 1 ). The enhanced luminescence is markedly diminished by the addition of Ca 2+ ( Fig. 2a ), indicating that Tb 3+ and Ca 2+ compete for access to a binding site or sites. Control liposomes with a matched amount of lipid ( Supplementary Fig. 1 ), but without ORAI1, produce only a modest enhancement of Tb 3+ luminescence ( Fig. 2a ). In this case, the luminescence probably results from direct excitation of Tb 3+ complexed with phosphatidylcholine (PC), and it can be explained by the known shift in the excitation spectrum of the Tb 3+ -PC complex relative to the excitation spectrum of unbound Tb 3+ (ref. 24 ). The Tb 3+ signal from control liposomes shows little or no competition by Ca 2+ ( Fig. 2a ), consistent with the very weak binding of Ca 2+ to PC [25] , [26] . There is no appreciable signal from Tb 3+ in buffer under these conditions [27] . 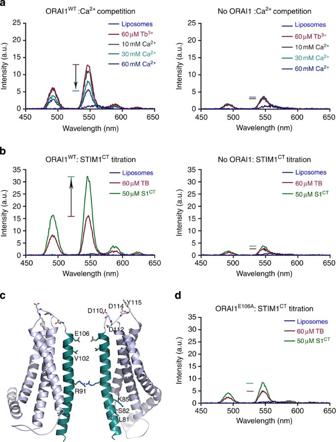Figure 2: Tb3+reports a STIM1-dependent conformational change in the ORAI1 channel. (a) Tb3+luminescence assay with equal amounts of liposomes containing ORAI1WTand control liposomes lacking ORAI (magenta curves in left and right panels, respectively). Sequential titration with 10–60 mM Ca2+reduces the Tb3+signal from ORAI1WTliposomes specifically. Representative of three experiments. (b) Tb3+luminescence from ORAI1WTchannels is enhanced upon titration of STIM1CT. The complete 10–50 μM STIM1CTtitration is presented inSupplementary Fig. 1a. Here the 50 μM STIM1CTcurve only is shown for clarity. Representative of eight experiments. (c) Cartoon representation of a cross-section of the human ORAI1 channel, on the basis of homology to theDrosophilaOrai channel, PDB accession number 4HKR. Only two subunits are depicted. The pore-lining TM1 helices from both subunits are coloured cyan, and residues mentioned in the text are highlighted in stick representation. (d) Tb3+luminescence of ORAI1E106Aliposomes in the same experiment asa. Equal amounts of ORAI1WTand ORAI1E106Aprotein were present in the assay, as verified by SDS–PAGE analysis and by amino acid analysis. Representative of four experiments. Ina,b, arrows indicate the direction of change of luminescence signal; ina,bandd, thin lines indicate the initial luminescence after addition of Tb3+and the final luminescence after titration with Ca2+or STIM1CT. Figure 2: Tb 3+ reports a STIM1-dependent conformational change in the ORAI1 channel. ( a ) Tb 3+ luminescence assay with equal amounts of liposomes containing ORAI1 WT and control liposomes lacking ORAI (magenta curves in left and right panels, respectively). Sequential titration with 10–60 mM Ca 2+ reduces the Tb 3+ signal from ORAI1 WT liposomes specifically. Representative of three experiments. ( b ) Tb 3+ luminescence from ORAI1 WT channels is enhanced upon titration of STIM1 CT . The complete 10–50 μM STIM1 CT titration is presented in Supplementary Fig. 1a . Here the 50 μM STIM1 CT curve only is shown for clarity. Representative of eight experiments. ( c ) Cartoon representation of a cross-section of the human ORAI1 channel, on the basis of homology to the Drosophila Orai channel, PDB accession number 4HKR. Only two subunits are depicted. The pore-lining TM1 helices from both subunits are coloured cyan, and residues mentioned in the text are highlighted in stick representation. ( d ) Tb 3+ luminescence of ORAI1 E106A liposomes in the same experiment as a . Equal amounts of ORAI1 WT and ORAI1 E106A protein were present in the assay, as verified by SDS–PAGE analysis and by amino acid analysis. Representative of four experiments. In a , b , arrows indicate the direction of change of luminescence signal; in a , b and d , thin lines indicate the initial luminescence after addition of Tb 3+ and the final luminescence after titration with Ca 2+ or STIM1 CT . Full size image Recombinant STIM1 CT in the range 10–50 μM further increases the Tb 3+ signal from ORAI1-containing liposomes ( Fig. 2b ). STIM1 CT does not enhance Tb 3+ luminescence by itself [27] , and STIM elicits little or no increase in the Tb 3+ signal from control liposomes ( Fig. 2b ). The effect of STIM1 might, in principle, reflect increased Tb 3+ binding to ORAI1, increased efficiency of energy transfer from protein to Tb 3+ , or decreased nonradiative decay of the Tb 3+ excited state and consequent increased Tb 3+ emission. Each possibility implies a conformational change in the vicinity of the Tb 3+ binding site or sites. There are two likely sites for Tb 3+ binding in the ORAI1 channel ( Fig. 2c ). The Drosophila Orai structure has shown that a ring of E178 residues (E106 residues in human ORAI1), projecting into the pore from transmembrane helix 1 (TM1), forms a lanthanide binding site [28] . In addition, electrophysiological studies of ORAI1 channel blockade by La 3+ have shown that acidic residues in the extracellular TM1–TM2 loops constitute an La 3+ binding site [29] . Each site is arguably situated within range for Y115-sensitized Tb 3+ luminescence. ORAI1 channels with an E106A substitution in the pore display very little Tb 3+ luminescence, and STIM1 CT causes only a small increase in the signal compared to the increase obtained with wild-type channels ( Fig. 2d ). This finding strongly suggests that the essential Ca 2+ -binding site formed by E106 side chains [30] , [31] , [32] , [33] makes a major contribution to Tb 3+ luminescence both in the absence and presence of STIM. However, D110A/D112A/D114A substitutions in the adjacent TM1–TM2 loop also decrease luminescence by ~50% ( Supplementary Fig. 1 ). The most plausible interpretation is that E106 is the primary Tb 3+ binding site for luminescence, and that negative charges in the TM1–TM2 loop increase binding to the E106 site by increasing the local concentration of Tb 3+ , but we do not rule out a contribution to luminescence from Tb 3+ bound to the TM1–TM2 loop. In either case, since the two possible binding sites are in close proximity, the STIM-induced increase in luminescence indicates a conformational change at or near E106 at the external entrance of the pore, triggered by STIM1 binding to the cytoplasmic face of the channel. STIM1 acts by engaging an ORAI1 N-terminal segment The ORAI1 conformational change depends on the amino (N)-terminal segment ORAI1(66–91), which is a site of physical interaction with STIM1 (refs 23 , 34 ). We introduced three mutations in ORAI1, 81 LSRAK 85 > 81 AARAE 85 , on the basis of cellular assays implicating the three targeted residues in STIM–ORAI activation [35] , [36] . These ‘LSK’ replacements substantially inhibit the STIM-elicited conformational change assessed with Tb 3+ ( Fig. 3a ; Supplementary Fig. 2a,b ). Conversely, the wild-type synthetic peptide ORAI1(66–91), added after STIM1 CT in the Tb 3+ luminescence assay with wild-type ORAI1, reverses the conformational change elicited by STIM1 ( Fig. 3b ). The same peptide has only a minimal effect on the luminescence of Tb 3+ bound to ORAI in the absence of STIM ( Supplementary Fig. 2c,d ), ruling out chelation of Tb 3+ by the peptide and nonspecific interference by the peptide with Tb 3+ binding to the channel. Direct measurement of STIM1 CT binding to synthetic ORAI1 N-terminal peptides, wild-type and mutant, confirms that the LSK replacements substantially reduce STIM-peptide affinity, as intended ( Supplementary Fig. 2e ). The N-terminal replacements do not interfere with STIM binding to recombinant ORAI1 channels in isolated yeast cell membranes ( Supplementary Fig. 2f ), a correlate of the finding that STIM–ORAI coclustering in mammalian cells depends mainly upon STIM interaction with the ORAI carboxy (C) terminus [37] , [38] , [39] . These findings imply that, following an initial STIM–ORAI interaction involving the ORAI C terminus, a second STIM–ORAI binding interaction involving the N-terminal segment of ORAI is necessary for the conformational change. 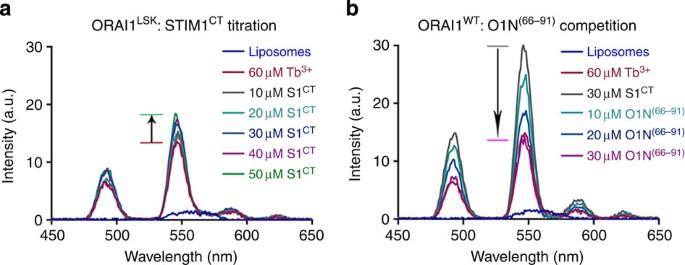Figure 3: An ORAI1 N-terminal segment is essential for the STIM1-mediated conformational change. (a) Tb3+luminescence from lipsomes reconstituted with ORAI1LSKon titration with 10–50 μM STIM1CT. Representative of four experiments. (b) The STIM1-dependent increase in Tb3+luminescence from ORAI1WTliposomes is reversed by titration with 10–30 μM synthetic ORAI1 N-terminal peptide. Sequential additions were Tb3+(magenta curve), STIM1CT(S1CT, grey curve), and synthetic ORAI1 N-terminal peptide (O1N(66–91)) to the final concentrations indicated. Representative of three experiments. Arrows ina,bindicate the direction of change of the luminescence signal. Figure 3: An ORAI1 N-terminal segment is essential for the STIM1-mediated conformational change. ( a ) Tb 3+ luminescence from lipsomes reconstituted with ORAI1 LSK on titration with 10–50 μM STIM1 CT . Representative of four experiments. ( b ) The STIM1-dependent increase in Tb 3+ luminescence from ORAI1 WT liposomes is reversed by titration with 10–30 μM synthetic ORAI1 N-terminal peptide. Sequential additions were Tb 3+ (magenta curve), STIM1 CT (S1 CT , grey curve), and synthetic ORAI1 N-terminal peptide (O1N (66–91) ) to the final concentrations indicated. Representative of three experiments. Arrows in a , b indicate the direction of change of the luminescence signal. Full size image The single replacement K85E in ORAI1 has been reported to result in a complete absence of STIM-dependent current in cells in response to Ca 2+ store depletion [35] , [40] , [41] , although STIM1 is able to gate the K85E ORAI1 channel when expressed as the active STIM1 CAD fragment, and particularly when the STIM1 CAD fragment is tethered to the channel [40] . In vitro the affinity of STIM1 for a synthetic K85E peptide is only modestly reduced compared with the affinity for wild-type peptide, and correspondingly STIM1 is able to cause a conformational change in the K85E channel, although with an apparent small shift in STIM1 concentration dependence ( Supplementary Fig. 3 ). The more profound deficit in the gating of the K85E channel in cells, compared with what we observe in vitro , might indicate that modulatory proteins interacting with the ORAI1 N-terminal segment control STIM-dependent gating in cells, as we have discussed elsewhere [42] . The same STIM–ORAI interaction underlies CRAC channel gating Analysis of this key STIM–ORAI interaction in parallel cellular assays links the conformational change in vitro to ORAI1 channel gating in cells. Overexpression of wild-type ORAI1 channels together with STIM1 results in a substantial Ca 2+ release-activated Ca 2+ (CRAC) current in HEK293T cells following store depletion, as expected, whereas overexpression of LSK ORAI1 channels with STIM1 does not ( Supplementary Fig. 4a–c ). Expression of the ORAI N-terminal peptide ORAI1(66–91) as a blue fluorescent protein (BFP) fusion protein does not interfere with ORAI1 recruitment into clusters following store depletion ( Fig. 4a ). The result is expected, since the STIM–ORAI interaction at the ORAI C terminus is intact. However, importantly, the peptide blocks CRAC current carried by endogenous ORAI1 channels in Jurkat T cells ( Fig. 4b–d ) and by overexpressed ORAI1 channels in HEK293T cells ( Fig. 4d ; Supplementary Fig. 4d–f ), indicating that the peptide has an inhibitory effect on the STIM–ORAI gating step. This blockade is a specific effect of the wild-type ORAI peptide, since expression of BFP fused to an ORAI N-terminal peptide with the LSK replacements does not block the current ( Fig. 4b–d ). These experiments reinforce recently published evidence that the STIM–ORAI N terminus interaction is required for channel gating by STIM in cells [40] , [41] , [43] , and add the key finding that the N-terminal ORAI1 peptide competes in vitro and in cells. The central conclusion is that the STIM–ORAI interaction required for the conformational change detected with Tb 3+ tracks closely with the interaction required for physiological STIM–ORAI communication in cells. 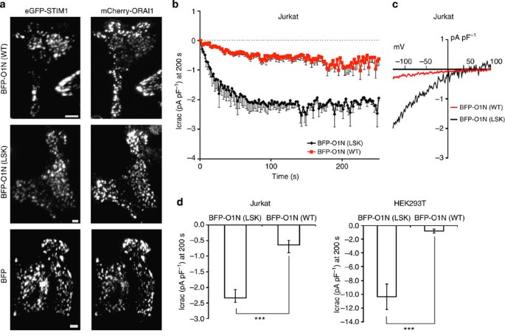Figure 4: An ORAI1 N-terminal segment is essential for the STIM1-mediated gating of ORAI1 in cells. (a) Single-channel TIRFM images of eGFP-STIM1 and mCherry-ORAI1 showing STIM–ORAI coclustering in HeLa cells co-expressing BFP-ORAI1(66–91) peptide (BFP-O1N (WT)), the corresponding LSK mutant (BFP-O1N (LSK)) or unmodified BFP. The images were acquired following treatment with thapsigargin. Scale bars, 1 μm. (b) Time course of CRAC current development (mean±SEM) in Jurkat T cells expressing only endogenous STIM1 and ORAI1, and transfected with BFP-O1N (WT) or BFP-O1N (LSK). (c) Typical current–voltage relationships recorded 200 s after break-in. (d) CRAC current density at 200 s (mean±SEM) showing a significant block of CRAC current due to expression of BFP-O1N (WT) peptide (for Jurkat cells,P=0.0065; for HEK293T cells,P=0.0086; by two-tailed Student’st-test). Numbers of cells used for analysis inbandd: Jurkat BFP-O1N (LSK), five; Jurkat BFP-O1N (WT), five; HEK293T BFP-O1N (LSK), six; HEK293T BFP-O1N (WT), five. Figure 4: An ORAI1 N-terminal segment is essential for the STIM1-mediated gating of ORAI1 in cells. ( a ) Single-channel TIRFM images of eGFP-STIM1 and mCherry-ORAI1 showing STIM–ORAI coclustering in HeLa cells co-expressing BFP-ORAI1(66–91) peptide (BFP-O1N (WT)), the corresponding LSK mutant (BFP-O1N (LSK)) or unmodified BFP. The images were acquired following treatment with thapsigargin. Scale bars, 1 μm. ( b ) Time course of CRAC current development (mean±SEM) in Jurkat T cells expressing only endogenous STIM1 and ORAI1, and transfected with BFP-O1N (WT) or BFP-O1N (LSK). ( c ) Typical current–voltage relationships recorded 200 s after break-in. ( d ) CRAC current density at 200 s (mean±SEM) showing a significant block of CRAC current due to expression of BFP-O1N (WT) peptide (for Jurkat cells, P =0.0065; for HEK293T cells, P =0.0086; by two-tailed Student’s t -test). Numbers of cells used for analysis in b and d : Jurkat BFP-O1N (LSK), five; Jurkat BFP-O1N (WT), five; HEK293T BFP-O1N (LSK), six; HEK293T BFP-O1N (WT), five. Full size image STIM1 repositions residue V102 in the pore-lining helix The Cu 2+ -phenanthroline crosslinking assay that we developed to map ORAI1 pore architecture [44] is an independent way to probe for a conformational change at the external entrance to the pore. Treatment with Cu 2+ -phenanthroline crosslinks pairs of cysteine side chains that are positioned suitably and is very sensitive to the local geometry of protein side chains, able to discriminate, for example, between the ‘a’ and ‘d’ positions in the hydrophobic core of a coiled coil [45] . We focused on V102, whose side chain projects into the pore one helical turn below E106. The valine > cysteine substitution needed for the crosslinking assay is conservative, replacing the valine side chain with a slightly smaller side chain of comparable hydrophobicity, and we verified that both the initial Tb 3+ luminescence signal of the V102C channel and the conformational change reported by a STIM-induced increase in Tb 3+ luminescence resemble those of the wild-type channel ( Fig. 5a ). 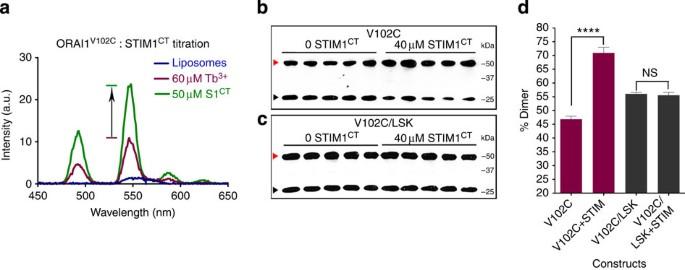Figure 5: STIM1-mediated conformational change at residue V102. (a) Tb3+luminescence from ORAI1V102Cshowing STIM1CT(S1CT)-dependent enhancement of the Tb3+signal comparable to that observed with ORAI1WT(Fig. 2b). Representative of three experiments. (b,c) Western blot analyses ofS. cerevisiae sec6-4vesicles expressing the Flag-tagged ORAI proteins V102C ORAI1 and LSK/V102C ORAI1, following Cu2+-phenanthroline crosslinking in the absence or presence of STIM1CT. Multiple samples were treated in parallel for each condition. Red and black arrowheads demarcate ORAI1 dimer and monomer bands, respectively. Representative of three to five experiments. (d) Fraction of ORAI1 in the dimer band (mean±SEM) from gels shown inb,c. ****P<0.0001 by two-tailed Student’st-test. No change was found in disulfide-linked dimer formation of FLAG-ORAI1LSK/V102Cfollowing STIM1CTtreatment (NS,P>0.05). Figure 5: STIM1-mediated conformational change at residue V102. ( a ) Tb 3+ luminescence from ORAI1 V102C showing STIM1 CT (S1 CT )-dependent enhancement of the Tb 3+ signal comparable to that observed with ORAI1 WT ( Fig. 2b ). Representative of three experiments. ( b , c ) Western blot analyses of S. cerevisiae sec6-4 vesicles expressing the Flag-tagged ORAI proteins V102C ORAI1 and LSK/V102C ORAI1, following Cu 2+ -phenanthroline crosslinking in the absence or presence of STIM1 CT . Multiple samples were treated in parallel for each condition. Red and black arrowheads demarcate ORAI1 dimer and monomer bands, respectively. Representative of three to five experiments. ( d ) Fraction of ORAI1 in the dimer band (mean±SEM) from gels shown in b , c . **** P <0.0001 by two-tailed Student’s t -test. No change was found in disulfide-linked dimer formation of FLAG-ORAI1 LSK/V102C following STIM1 CT treatment (NS, P >0.05). Full size image We then expressed V102C ORAI channels in Saccharomyces cerevisiae and carried out the crosslinking directly in the isolated membrane fraction, without solubilization and purification of the ORAI channels. After crosslinking in the absence of STIM1, a fraction of V102C channel subunits migrates as the crosslinked dimer on a nonreducing SDS–polyacrylamide gel [44] . STIM1 CT at concentrations that are effective in the Tb 3+ luminescence assay increases crosslinking at V102C ( Fig. 5b,d ), indicating that STIM1 causes a physical rearrangement at V102 in the wild-type channel. The increased crosslinking is dependent on STIM interaction with the N terminus of ORAI, since there is no STIM-dependent increase in crosslinking in the case of the LSK/V102C channel ( Fig. 5c,d ). These findings reinforce the principal conclusion from the Tb 3+ assay—that STIM interaction with the ORAI N-terminal region triggers a conformational change near the external mouth of the pore in the wild-type channel. The segment L95–V102 limits ion flux in the closed channel The observation that STIM-elicited movements extend to the vicinity of E106 and V102 suggested that the wild-type ORAI1 channel might have an external gate at V102 or in the adjacent nonpolar region of the pore [21] , [46] , contrary to a recent consensus view that places the sole channel gate at the cytoplasmic end of TM1 or in the N-terminal cytoplasmic extension of TM1 (refs 10 , 28 , 41 , 47 ). To assess the possible presence of a barrier to ion flux in the nonpolar region of the pore, we engineered an ORAI1(Δ1–88/R91G) channel that lacks any semblance of the proposed internal gate ( Fig. 6a ). The entire N-terminal region ORAI1(1–88) was replaced by a short peptide, MASSYTAPQPGLG–, with no pronounced propensity to form an α-helix, and R91 was replaced by glycine, leaving only the nonpolar segment from L95–V102 as a potential barrier to ion permeation. 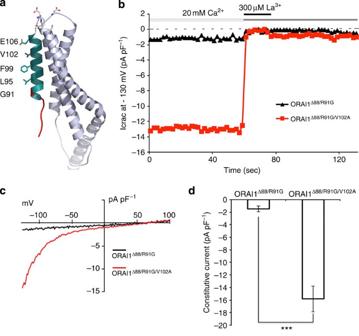Figure 6: The nonpolar region of the ORAI1 pore is a barrier to ion permeation. (a) Cartoon representation of the truncated ORAI1 constructs, on the basis of homology to theDrosophilaOrai channel, PDB accession number 4HKR. A single monomer is depicted, with the TM1 helix highlighted in cyan, the ORAI1 N-terminal residues 1–88 replaced by the 13-residue segment MASSYTAPQPGLG– shown as a red unstructured line, and the position where R91 is replaced by glycine marked by the red helical face. E106, V102 and nonpolar residues F99 and L95 in the two helical turns below V102 are shown in stick representation. V102 is mutated to alanine in the ORAI1Δ1–88/R91G/V102Aconstruct. (b) Current density at −130mV in representative HEK293T cells transfected with ORAI1Δ1–88/R91G(black curve) or with ORAI1Δ1–88/R91G/V102A(red curve). La3+was applied as an ORAI1 channel blocker to estimate leakage current, which was taken as the minimum inward current observed in each cell during La3+application. The duration of local La3+application is marked as a black line; the grey line denotes continuing exposure to declining concentrations of La3+during the time that La3+diffuses into the bulk solution. (c) Typical current–voltage relationship of the La3+-sensitive component of current. The constitutive ORAI1Δ1–88/R91G/V102Acurrent reverses at a potential positive to +50 mV, indicating an ion selectivity that differs from that of full-length V102A ORAI1, and shows prominent inward current only at rather negative membrane potentials. (d) Average constitutive current density (mean±SEM) differs significantly for ORAI1Δ1–88/R91G/V102Achannels and ORAI1Δ1–88/R91Gchannels (P=0.00014 by two-tailed Student’st-test). Numbers of cells used for analysis: ORAI1Δ1–88/R91G, six; ORAI1Δ1–88/R91G/V102A, 10. Figure 6: The nonpolar region of the ORAI1 pore is a barrier to ion permeation. ( a ) Cartoon representation of the truncated ORAI1 constructs, on the basis of homology to the Drosophila Orai channel, PDB accession number 4HKR. A single monomer is depicted, with the TM1 helix highlighted in cyan, the ORAI1 N-terminal residues 1–88 replaced by the 13-residue segment MASSYTAPQPGLG– shown as a red unstructured line, and the position where R91 is replaced by glycine marked by the red helical face. E106, V102 and nonpolar residues F99 and L95 in the two helical turns below V102 are shown in stick representation. V102 is mutated to alanine in the ORAI1 Δ1–88/R91G/V102A construct. ( b ) Current density at −130mV in representative HEK293T cells transfected with ORAI1 Δ1–88/R91G (black curve) or with ORAI1 Δ1–88/R91G/V102A (red curve). La 3+ was applied as an ORAI1 channel blocker to estimate leakage current, which was taken as the minimum inward current observed in each cell during La 3+ application. The duration of local La 3+ application is marked as a black line; the grey line denotes continuing exposure to declining concentrations of La 3+ during the time that La 3+ diffuses into the bulk solution. ( c ) Typical current–voltage relationship of the La 3+ -sensitive component of current. The constitutive ORAI1 Δ1–88/R91G/V102A current reverses at a potential positive to +50 mV, indicating an ion selectivity that differs from that of full-length V102A ORAI1, and shows prominent inward current only at rather negative membrane potentials. ( d ) Average constitutive current density (mean±SEM) differs significantly for ORAI1 Δ1–88/R91G/V102A channels and ORAI1 Δ1–88/R91G channels ( P =0.00014 by two-tailed Student’s t -test). Numbers of cells used for analysis: ORAI1 Δ1–88/R91G , six; ORAI1 Δ1–88/R91G/V102A , 10. Full size image We recorded whole-cell currents under voltage-clamp and used a standard test for CRAC/ORAI current, block by 300 μM La 3+ , to determine whether the truncated ORAI1(Δ1–88/R91G) channel carries constitutive current. A corresponding truncated channel with the V102A substitution, which is known to result in a constitutively conducting channel [21] , [41] , served as a control. The two truncated ORAI1 proteins were expressed at similar levels at the cell surface as judged by immune staining for an HA-tag incorporated into the second extracellular loop [31] ( Supplementary Fig. 5 ). Cells expressing the truncated V102A channel exhibited a substantial constitutive current, with typical current densities in the range 10–20 pA pF −1 ( Fig. 6b–d ), demonstrating that the truncated channels have no inherent defect in assembly or in their ability to conduct current. In contrast, cells expressing the truncated ‘wild-type’ channel exhibited only small constitutive currents, with current densities ~1 pA pF −1 ( Fig. 6b–d ). Interestingly, cells expressing an ORAI1(Δ1–64) channel also exhibited the small constitutive current under our conditions ( Supplementary Fig. 6 ), and therefore the current is not simply correlated with the absence or presence of the ORAI N-terminal cytoplasmic helices. We cannot say at present whether this small constitutive current is intrinsic to the channel or is an artifact of our experimental conditions, but, given its small amplitude in comparison with the current carried by the corresponding V102A channel ( Fig. 6b–d , Supplementary Fig. 6 ), we conclude that a truncated ORAI1 channel lacking any internal gate retains a barrier to ion flux. We conducted a further series of experiments that included the STIM1-gated channel ORAI1(Δ1–64) and its V102A variant ( Supplementary Fig. 6 ). When we expressed either the truncated wild-type channel or the ORAI1(Δ1–64) channel together with STIM1, and depleted ER Ca 2+ stores, only cells expressing ORAI1(Δ1–64) showed development of CRAC current ( Supplementary Fig. 6a ). This result confirms the requirement for the ORAI1 N-terminal segment in channel gating by STIM1. When the ORAI proteins were expressed without STIM, there were signature differences between the I–V curve of the truncated V102A channel ( Fig. 6c and Supplementary Fig. 6c , right) and those of the V102A ORAI1(Δ1–64) ( Supplementary Fig. 6c , right) and full-length V102A ORAI1 channels [21] , [41] that will require separate investigation. However, the constitutive current in cells expressing the truncated wild-type ORAI1 channel was small, whether the comparison was with the STIM1-gated CRAC current, the constitutive current of the truncated V102A ORAI1(Δ1–88/R91G) channel or the constitutive current of a V102A ORAI1(Δ1–64) channel ( Supplementary Fig. 6 ). The second series of experiments therefore reinforces our conclusion that the nonpolar segment from L95–V102 of the ORAI1 pore-lining helix is a barrier to ion permeation through the closed wild-type ORAI1 channel. SCID mutation R91W prevents the ORAI1 conformational change An R91W replacement in the N-terminal segment of ORAI1 causes a rare hereditary severe combined immunodeficiency (SCID) syndrome [22] . The R91W channel coclusters with STIM1 following Ca 2+ store depletion [38] , [39] , [41] , but it produces no CRAC current [22] , [38] , [41] . Because R91 is positioned in the linear sequence between the N-terminal STIM-binding peptide and TM1, we explored the physical and functional interactions of STIM1 CT with the R91W channel using in vitro binding and Tb 3+ luminescence assays. A sucrose gradient flotation assay demonstrates that STIM1 binds R91W ORAI1 channels in isolated yeast cell membranes ( Supplementary Fig. 7a ), again consistent with a primary STIM interaction that engages the ORAI C terminus [37] , [38] , [39] , and consistent with FRET experiments that have directly probed the STIM1–R91W ORAI1 interaction in mammalian cells [38] , [39] , [41] . Further, there is no intrinsic deficit in STIM1 binding to a synthetic R91W ORAI1 N-terminal peptide, since recombinant STIM1 CT binds to synthetic wild-type ORAI1(66–91) with K d ~10 μM and to the synthetic R91W peptide with similar affinity ( Supplementary Fig. 7b ). However, STIM1 CT fails to increase the luminescence of Tb 3+ bound to the R91W ORAI1 channel ( Fig. 7a,b ), indicating that the mutation interferes with the STIM1-dependent conformational change. STIM1 CT binding to the R91W/V102C channel likewise has no effect on V102C crosslinking ( Fig. 7c,d ), reinforcing the result of the Tb 3+ assay. Thus, the specific deficit in R91W ORAI1 is that STIM1 does not elicit the extensive conformational change observed in the wild-type channel, most likely because the ring of tryptophan residues stabilizes the N-terminal peptide in a configuration that cannot interact productively with STIM1. 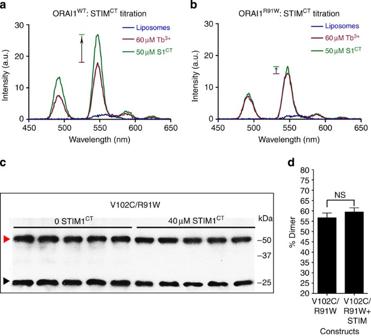Figure 7: ORAI1R91Wshows no STIM1-dependent enhancement of Tb3+luminescence. (a) The positive control, ORAI1WTreconstituted into liposomes, shows a substantial increase in Tb3+luminescence upon addition of STIM1CT(S1CT). (b) Titration of 10–50 μM STIM1CTinto the sample with ORAI1R91Wreconstituted into liposomes has a negligible effect on luminescence. For clarity, only the 50 μM STIM1CTcurves are shown. The ORAI1WTand ORAI1R91Wsamples contained equal amounts of ORAI protein. Representative of four experiments. (c) Western blot analysis ofS. cerevisiae sec6-4vesicles expressing Flag-tagged R91W/V102C ORAI1, following Cu2+-phenanthroline crosslinking in the absence or presence of STIM1CT. Red and black arrowheads demarcate ORAI1 dimer and monomer bands, respectively. Representative of four experiments. (d) Fraction of ORAI1 in the dimer band (mean ±SEM) from the gels shown inc. No change was found in disulfide-linked dimer formation of FLAG-ORAI1V102C/R91Wfollowing STIM1CTtreatment (NS,P>0.05 by two-tailed Student’st-test). Representative of four experiments. Figure 7: ORAI1 R91W shows no STIM1-dependent enhancement of Tb 3+ luminescence. ( a ) The positive control, ORAI1 WT reconstituted into liposomes, shows a substantial increase in Tb 3+ luminescence upon addition of STIM1 CT (S1 CT ). ( b ) Titration of 10–50 μM STIM1 CT into the sample with ORAI1 R91W reconstituted into liposomes has a negligible effect on luminescence. For clarity, only the 50 μM STIM1 CT curves are shown. The ORAI1 WT and ORAI1 R91W samples contained equal amounts of ORAI protein. Representative of four experiments. ( c ) Western blot analysis of S. cerevisiae sec6-4 vesicles expressing Flag-tagged R91W/V102C ORAI1, following Cu 2+ -phenanthroline crosslinking in the absence or presence of STIM1 CT . Red and black arrowheads demarcate ORAI1 dimer and monomer bands, respectively. Representative of four experiments. ( d ) Fraction of ORAI1 in the dimer band (mean ±SEM) from the gels shown in c . No change was found in disulfide-linked dimer formation of FLAG-ORAI1 V102C/R91W following STIM1 CT treatment (NS, P >0.05 by two-tailed Student’s t -test). Representative of four experiments. Full size image Analysis of ORAI channel gating has been hindered because STIM-dependent activation of ORAI channels is not amenable to standard electrophysiological approaches, such as measuring gating currents or determining the kinetics of single-channel openings. Here we have shown that recombinant STIM1 gates Ca 2+ flux through the purified recombinant ORAI1 channel reconstituted into liposomes. Taking advantage of this reconstituted system, and the intrinsic ability of Tb 3+ to bind at the key Ca 2+ -binding site in the channel pore, we have been able to observe a STIM1-triggered movement near the external mouth of the channel, occurring over the same concentration range of STIM1 that elicits Ca 2+ flux. The use of Tb 3+ as a probe avoided any bias associated with the introduction of mutations or covalent labels, and allowed us to monitor gating of the unmodified wild-type channel. We have provided corroborating biochemical evidence that STIM1 also elicits movement at the adjacent pore residue V102. Finally, in complementary electrophysiological experiments, we have located an external barrier to Ca 2+ flux in the section of the pore lined by V102 and adjacent nonpolar side chains. Our data offer the first direct insight into the gating mechanism of an ORAI channel. The selectivity of CRAC channels for Ca 2+ over Na + results from Ca 2+ binding at a site in the pore [19] , [48] . The binding site was mapped to E106 in ORAI1 by the demonstration that an E106D substitution reduces ion selectivity and shifts the concentration dependence of Ca 2+ block of Na + current through the channel [20] , [30] , [31] , [32] , [33] . Disulfide crosslinking of E106C ORAI1 monomers confirmed that the E106 side chains are in proximity and thus positioned to form a Ca 2+ -binding site [44] , a conclusion later confirmed for the corresponding E178 residues in the high-resolution Drosophila Orai structure [28] . The Tb 3+ luminescence changes reported here suggest that a repositioning of the E106 residues is an integral part of ORAI1 channel gating. The position of the gate in ORAI channels has been a matter of debate. A widely favoured view has been that the ORAI1 channel gate is located at the cytoplasmic end of TM1 or in the N-terminal cytoplasmic extension of TM1 (refs 10 , 28 , 41 , 47 ), with channel opening arising from bending of the TM1 helices at the conserved glycine residues G98 (ref. 47 ) or from flexion of the helices aided by the five serine, threonine and glycine residues between S89 and G98 (ref. 28 ). The experimental evidence for an internal gate is indirect, however, based mainly on the reversible block produced by Cd 2+ binding or by disulfide crosslinking at the cysteine residues of an R91C channel [29] , [47] . We submit that the latter observations show only that the segments flanking R91 in individual ORAI monomers, which are somewhat flexible [44] , can approach each other. They do not imply that the cytoplasmic segments of the closed wild-type channel remain in a fixed helix bundle resembling that in the Drosophila Orai crystal structure. In contrast to the view outlined above, McNally et al . [21] demonstrated clearly that there is a physical gate external to G98C in the G98C/E106D ORAI1 channel that restricts access of a methanethiosulfonate reagent, applied extracellularly, to the introduced G98C cysteine when the channel is closed . Although ‘substituted cysteine accessibility’ [49] has been a standard method for locating the gate in other channels, the evidence for G98C/E106D ORAI1 did not lead to a consensus that there is an external gate in the wild-type ORAI1 channel, perhaps because a local narrowing of the ORAI channel that hinders the passage of methanethiosulfonate reagent need not hinder the flux of smaller permeant ions [29] , or because several G98X mutants and the E106D mutant show alterations in channel activation and other pore properties [43] , [47] , [50] . Here we have provided direct evidence that a barrier to ion flux is present in the wild-type ORAI1 channel pore and maps to an external region of the pore-lining helix that moves when STIM1 gates the channel. Clearly the above considerations do not rule out the possibility that the ORAI1 channel has an internal gate. STIM1 binds to the cytoplasmic segments ORAI1(66–91) (refs 23 , 34 ) and might thereby constrain them in a position more conducive to ion flux. Since the same binding interaction initiates the conformational rearrangement in the external region of the pore, a direct demonstration that there is an internal gate would imply a concerted gating movement extending along the entire length of the pore-lining helices. The evidence for a gate near V102 dovetails with earlier findings that the V102C, V102A, V102G, V102S and V102T ORAI1 channels carry constitutive current in the absence of STIM1 (refs 21 , 41 ). In the simplest scenario, replacement of the V102 side chain with any of these smaller side chains results in a leaky gate, in a channel whose overall conformation is that of the resting wild-type channel. This scenario is supported by in silico calculations indicating that the barrier to ion flux is lower in the Drosophila V174A Orai channel (corresponding to V102A ORAI1) than in the wild-type channel, whereas there is no substantive difference in the protein conformations [46] . It also gains support from our finding that V102C ORAI1 channels exhibit an increase in Tb 3+ luminescence upon STIM1 CT binding, rather than displaying the constitutively elevated luminescence expected of preactivated channels, though we cannot say from measurement of this single variable that the conformation of the V102C channel before STIM1 CT binding is identical to that of the wild-type channel. A subtext is that, on current evidence, the V102X channels cannot be taken as a faithful model of the physiologically gated wild-type channel. The Tb 3+ luminescence experiments clarify the defect of the SCID mutant R91W ORAI1 channel, whose failure to conduct Ca 2+ formed part of the original evidence pinpointing ORAI1 as a CRAC channel subunit [22] . The close packing of the six tryptophan side chains in the crystal structure of K163W Drosophila Orai [28] and the fact that the R91W/V102C ORAI1 channel is nonconducting [21] leave little doubt that the tryptophan side chains occlude the pore. However, the primary defect of the R91W ORAI1 mutant is in channel gating. Our findings using the reconstituted STIM–ORAI system animate views of pore architecture derived from electrophysiology [20] , [21] , [29] , [30] , [31] , [32] , [33] , protein biochemistry [44] and the recent structure of the Drosophila Orai channel [28] . Further studies with purified STIM and ORAI proteins will be an important complement to cellular studies for insights into ORAI channel gating, modulation and inactivation. Recombinant protein purification Wild-type ORAI1 for biochemical and biophysical studies in vitro was a cysteineless human ORAI1 65–301 (N223A), with 6xHis and FLAG tags and a TEV protease cleavage site preceding the ORAI1 coding sequence, expressed from a pBEVY-GU plasmid [51] under control of its GAL1 promoter. Specified mutants were produced using the Quikchange site-directed mutagenesis kit (Agilent). Plasmids were introduced into S. cerevisiae strain NY17 (MAT a , ura3 - 52 , sec6 - 4 ) by electroporation using a Micropulser (Bio-Rad) with standard pulse settings for yeast cells [52] . S. cerevisiae strain NY17 (MAT a , ura3-52 , sec6-4 ) cells were grown to mid-log phase at 25 °C in uracil-deficient synthetic complete medium containing glucose (SC-URA/glucose medium). Protein expression was induced in SC-URA/galactose medium at the nonpermissive temperature, 37 °C, to cause intracellular accumulation of newly synthesized ORAI1 in 100-nm vesicles in transit to the plasma membrane. The cells were collected at 4,000 g for 5 min at 4 °C and resuspended in 50 mM Tris-Cl, pH 7.5, 150 mM NaCl and Protease Inhibitor Cocktail (Roche). Cells were lysed by adding one volume of acid-washed 400-μm glass beads and vortexing with 1 min on-off cycles, the lysate was cleared of cell debris and nuclei by pelleting at 1,000 g for 15 min at 4 °C, and a membrane fraction containing the 100-nm vesicles was collected by centrifugation at 167,000 g for 30 min at 4 °C and resuspended in 50 mM Tris-Cl, pH 7.5, 150 mM NaCl. This ‘vesicle fraction’ was used for disulfide crosslinking and membrane flotation assays. For purification of ORAI proteins, S. cerevisiae cells grown as above were collected and resuspended in lysis buffer consisting of 50 mM HEPES-Na pH 7.5, 300 mM NaCl, with Protease Inhibitor Cocktail. Cells were lysed using a microfluidizer M-110P (Microfluidicscorp), unlysed cells and debris were removed by centrifugation at 4,000 g , and membranes were pelleted by centrifugation at 100,000 g . The membrane pellet was resuspended in lysis buffer with 1% decyl maltoside (Affymetrix), and solubilized proteins were fractionated by cobalt-affinity chromatography on Talon affinity resin (Clontech), where the recombinant ORAI proteins eluted at 250 mM imidazole, and size-exclusion chromatography on a Superose 6 column (GE) in the course of which NaCl concentration was reduced to 150 mM. Proteins were concentrated to 30 mg ml −1 in 50 mM Tris-Cl, pH 7.5, 150 mM NaCl, 0.12% decyl maltoside. 6xHis-STIM1 CT was mouse STIM1 cytoplasmic domain (residues 233–685) expressed in Escherichia coli BL21(DE3) cells and purified by Ni-NTA affinity chromatography and size-exclusion chromatography as described [23] . The purification was completed within 5 h from lysis to maximize the yield of active protein. ORAI1 reconstitution Purified ORAI1 was reconstituted into liposomes consisting of PC and phosphatidylserine (PS) in a molar ratio of 80:20. All liposome preparations used in an experiment were adjusted to similar lipid concentrations on the basis of light scattering at 600 nm and staining with a lipid-soluble dye. The incorporation of equal amounts of different ORAI proteins into the liposomes used for each individual experiment was confirmed by analysis on SDS–polyacrylamide gels and, in selected cases, by amino acid analysis at the W.M. Keck Foundation Biotechnology Resource Laboratory, Yale University. In more detail, the lipids 1-hexadecanoyl-2-(9Z-octadecenoyl)- sn -glycero-3-phosphocholine (PC; Avanti Polar Lipids) and 1-palmitoyl-2-oleoyl- sn -glycero-3-phospho-L-serine (PS; Avanti Polar Lipids) in chloroform were mixed in a molar ratio of 80:20 and dried under a stream of argon and then overnight under vacuum. The dried lipids were rehydrated for 3–4 h in 50 mM Tris-Cl pH 7.5, 150 mM NaCl, with repeated vortexing. Purified ORAI1 protein (or a corresponding amount of buffer for control liposomes lacking ORAI1) was added at a protein:lipid ratio (w/w) of 1:20 and incubated for 1 h. Detergent was removed from the proteoliposomes with Bio-Beads SM-2 (Bio-Rad). Liposomes were monitored by light scattering at 600 nm. To compare total lipids present in different liposome preparations, the samples were incubated with the lipophilic carbocyanine dye DiD (Life Technologies) for 10 min, washed twice by centrifugation at 167,000 g , and quantified using absorbance at 665 nm. An example of these measurements is shown in Supplementary Fig. 1e . Ca 2+ flux assay For the Ca 2+ flux assays, PC, PS and L-α-phosphatidylinositol-4-phosphate (PI4P; Avanti Polar Lipids) were included in the liposomes at a ratio of 75:20:5. The buffer used for liposome formation was 50 mM Tris-Cl pH 7.5, 10 mM KCl, containing 2–5 mM CaCl 2 . Following formation of proteoliposomes, five freeze-thaw cycles (between −196 °C and 37 °C) were performed. The Ca 2+ flux assay buffer was 50 mM Tris-Cl pH 7.5, 150 mM KCl, 2 μM Fura-2. All reagents used during the final fluorimetric analysis, including purified recombinant STIM1 CT and liposomes, were passed through BAPTA-polystyrene (Calcium Sponge S; Life Technologies) to remove traces of free Ca 2+ . A 130-μl aliquot of liposome suspension was transferred to a microcuvette, and excitation spectra were recorded from 300–450 nm at a fixed emission wavelength of 510 nm, initially and following sequential additions of purified STIM1 CT into the cuvette to final concentrations 20–100 μM as indicated. Finally, digitonin was added to verify that the liposomes contained releasable Ca 2+ . Tb 3+ luminescence assay Liposome suspension (130 μl) was excited at 280 nm using a pulsed xenon excitation source in a QM40 spectrofluorometer (Photon Technology International). Sensitized Tb 3+ emission, gated at 200 μs to discriminate Tb 3+ luminescence from light scattering and endogenous fluorescence, was recorded from 450–650 nm with the slit width set at 12 nm. Sequential additions of Tb 3+ to final concentration 60 μM, and then of Ca 2+ or purified STIM1 CT or synthetic ORAI1(66–91) peptide, were made as specified. ORAI1 crosslinking Copper phenanthroline (CuP) crosslinking was carried out as described [44] with some modifications. Yeast sec6-4 vesicles in 50 mM Tris-Cl pH 7.5, 150 mM NaCl, 0.3 mM DTT, at a total protein concentration of 1–1.5 mg ml −1 as measured by NanoDrop spectrophotometer ND-1000 (NanoDrop), were distributed in aliquots of 10 μl per well in a round-bottom 96-well plate. STIM1 CT was added in 10 μl buffer to the specified final concentration, with an equivalent addition of buffer alone to control samples. Samples were incubated for 10 min at room temperature, then treated with 1 mM CuP for 10 min at room temperature; quenched with a stop solution containing 50 mM Tris-Cl pH 7.4, 20 mM N-ethylmaleimide and 20 mM EDTA; mixed with 5 × nonreducing SDS loading buffer; and heated at 55 °C for 15 min. The level of ORAI1 crosslinking was analysed by SDS–PAGE using 4–12% NuPAGE Bis-Tris gels (Invitrogen) and immunoblotting for ORAI1 monomer and dimer. Immunoblotting was performed using anti-FLAG-M2 and HRP-labelled secondary antibodies (Sigma), and the blots were developed using ECL substrate (Perkin Elmer). Relative intensities of monomer and dimer bands in images of the blots were quantified using ImageJ software (National Institutes of Health). STIM1 binding to ORAI1 channels The membrane flotation assay is based on the assay used previously with Pichia pastoris membranes [23] . Yeast sec6-4 vesicles (38 μl at 1–1.5 mg ml −1 total protein concentration) were incubated with purified STIM1 CT (2 μl of an 80 μM stock) or dilution buffer for 1 h at 4 °C. Each sample was overlaid sequentially with 400 μl of 80% (w/v) sucrose, 3 ml of 60% (w/v) sucrose and 400 μl of 10% (w/v) sucrose; and the samples were centrifuged at 100,000 g for 16 h at 4 °C in an SW50.1 Ti rotor (Beckman Coulter). Five 750-μl fractions were collected from top to bottom of the gradient, and a 20-μl aliquot of each fraction was analysed by electrophoresis on a 4–12% Bis-Tris NuPAGE gradient gel (Invitrogen) and western blotting with anti-FLAG-M2 monoclonal antibody (Sigma) for FLAG-tagged ORAI1 and anti-STIM1 antibody (Cell Signaling Technology) for 6xHis-STIM1 CT . STIM1 binding to synthetic ORAI1 peptide Synthetic fluorescein-labelled ORAI1(66–91) peptides, incorporating an N-terminal fluorescein-thiocarbamyl-6-aminohexanoyl residue, were synthesized at the Tufts University Core Facility. ORAI peptide sequences used in this study were LNEHSMQALSWRKLYLSRAKLKASSR (wild-type), LNEHSMQALSWRKLYAARAELKASSR (LSK variant), LNEHSMQALSWRKLYLSRAELKASSR (K85E variant), and LNEHSMQALSWRKLYLSRAKLKASSW (R91W variant). Peptides were dissolved in dimethylsulfoxide, then diluted to 280 nM in 50 mM Tris-Cl pH 7.5, 150 mM NaCl. STIM1 CT was titrated into the cuvette containing labelled peptide, and the polarization of fluorescein-peptide fluorescence was measured as a function of added STIM1 CT . STIM1 and ORAI1 expression in mammalian cells Wild-type full-length human ORAI1 1–301 and its LSK mutant, with an eGFP tag at the C terminus, were expressed together with untagged full-length human STIM1 in the experiments of Supplementary Fig. 4a–c . The BFP–ORAI1(66–91) fusion construct in the pTagBFP-C vector (Evrogen) was expressed alone in the experiments of Fig. 4b–d , and together with expression constructs for eGFP-STIM1 in pCMV6-XL5 vector and mCherry-ORAI1 in MO91 vector [53] in the experiments of Fig. 4a and Supplementary Fig. 4d–f . A corresponding BFP–ORAI1(66–91) fusion protein with the LSK substitutions and BFP expressed from the unmodified vector served as controls. The truncated ORAI1 proteins of Fig. 6 and Supplementary Figs 5 and 6 were derived from human ORAI1(89–301) with the N-glycosylation site mutation N223A and with an HA-tag in the second extracellular loop [31] . The sequence N-terminal to residue 89 was replaced by MASSYTAPQPGLG–, and arginine-91 was replaced by glycine. The sequence engineered into the second extracellular loop between ORAI1 residues 206 and 207 was VDGSGSYPYDVPDYAGSGSTR, consisting of the HA-tag YPYDVPDYA flanked by short linker sequences [31] . Another pair of constructs encoded the corresponding HA-tagged ORAI1(Δ1–64) proteins. The proteins were expressed from a pcDNA3.1(+) vector (Life Technologies) under control of the human cytomegalovirus (CMV) promoter. In the experiments of Supplementary Fig. 6a , ORAI1 proteins were expressed together with eGFP-STIM1. Total internal reflection fluorescence microscopy A HeLa cell line stably expressing eGFP-STIM1 and mCherry-ORAI1 (ref. 53 ) was maintained at 37 °C under 10% CO 2 in Dulbecco’s Modified Eagle’s medium (DMEM; HyClone media, Thermo) containing 10% heat-inactivated FBS. The cells were transfected with expression plasmid for wild-type or LSK mutant BFP-ORAI1(66–91) or for BFP, as indicated, using Lipofectamine-2000 (Life Technologies) according to the manufacturer’s instructions. Cells were stimulated with thapsigargin to deplete ER Ca 2+ stores prior to image acquisition. Total internal reflection fluorescence microscopy (TIRFM) was performed using Nikon CFI Apo objectives ( × 60, 1.45 NA) mounted on a Ti-Eclipse inverted microscope with Perfect Focus System (PFS; Nikon). Images were acquired using a Coolsnap HQ2 monochrome CCD camera (Photometrics). Electrophysiology HEK293T cells cultured at 37 °C under 10% CO 2 in DMEM containing 10% heat-inactivated FBS were transfected with the specified expression plasmids using Lipofectamine-2000 (Life Technologies). Transfected cells were plated on poly-L-lysine (Sigma) treated 25 mm glass coverslips in DMEM containing 10% heat-inactivated FBS and 50 μM 2-mercaptoethanol. Jurkat T cells were cultured at 37 °C under 10% CO 2 in RPMI (HyClone media, Thermo) containing 10% heat-inactivated FBS and electroporated using the NEON transfection system (Life Technologies). The combinations of expression plasmids used in particular experiments are detailed in ‘STIM1 and ORAI1 expression in mammalian cells’. To identify transfected cells in the experiments of Fig. 6 and Supplementary Fig. 6b–d , pMax-GFP vector (Amaxa) was co-transfected with the ORAI1 variants, and only green fluorescent cells were chosen for recording. In the experiments of Supplementary Fig. 6a , the cells were co-transfected with ORAI1 and eGFP-STIM1 expression plasmids, and green fluorescent cells were chosen for recording. Whole-cell patch-clamp recordings were performed at 21–25 °C. Micropipettes with resistance 2.8–3.2 MΩ were pulled and fire-polished. To reduce electrode capacitance, pipettes were siliconized with Sigmacote (Sigma) immediately before use. Membrane currents were acquired with an EPC-9 patch-clamp amplifier (HEKA). Voltage ramps of 200-ms duration spanning a range of −150 to +100 mV were delivered from a holding potential of 0 mV at a rate of 0.5 Hz. Pipette and cell capacitance were electronically cancelled before each voltage ramp. Currents were filtered at 2.9 kHz and digitized at a sampling rate of 10 kHz. For display, currents were digitally filtered offline at 1 kHz. All voltages were corrected for a liquid-junction potential of −10 mV between internal and bath solutions. Current amplitudes at −130 mV from individual ramps were used to follow the temporal development of currents, which are graphed for representative cells or as averaged data (mean±s.e.m.) for each condition. The external solution was 120 mM NaCl, 2 mM MgCl 2 , 20 mM CaCl 2 , 10 mM TEA-Cl, 10 mM glucose, 10 mM HEPES, pH 7.2 with NaOH. The pipette solution for measurements of STIM-mediated CRAC current contained 0.05 mM inositol 1,4,5-trisphosphate (InsP 3 ), 50 nM thapsigargin, 140 mM Cs glutamate, 3 mM MgCl 2 , 12 mM EGTA, 10 mM HEPES, pH 7.2 with CsOH. For the experiments with truncated ORAI1 channels and ORAI1(Δ1–64) channels, other than the experiments in Supplementary Fig. 6a , the pipette solution contained neither InsP 3 nor thapsigargin, and EGTA concentration was 1.2 mM to minimize the passive depletion of ER Ca 2+ stores during the brief period of recording. Except in the case of constitutive current measurements, the background current measured in the first voltage ramp after break-in was subtracted. To isolate the La 3+ -blockable component of current, an external solution containing 300 μM LaCl 3 was perfused locally during recording, and the minimum inward current observed during La 3+ application was taken as background current. In the I–V curves of Fig. 6c and Supplementary Fig. 6b,c and the histograms of Fig. 6d and Supplementary Fig. 6d , this background was subtracted. Flow cytometry To quantitate the surface expression of the HA-tagged truncated ORAI proteins, transfected HEK293T cells were detached carefully using Hanks’-based enzyme-free cell dissociation buffer (Gibco), washed twice and resuspended in PBS/0.1% bovine serum albumin. The cells were stained with anti-HA antibody conjugated to AlexaFluor 647 and analysed using a FACSCalibur flow cytometer (BD Biosciences). Dead cells were excluded from the analysis on the basis of their uptake of propidium iodide. Statistical analysis and curve fitting Differences in CRAC current density and in ORAI dimer:monomer ratios in the crosslinking experiments were analysed by two-tailed Student’s t -test. STIM–ORAI peptide binding data were fitted to a single-site binding model using GraphPad Prism. How to cite this article : Gudlur, A. et al . STIM1 triggers a gating rearrangement at the extracellular mouth of the ORAI1 channel. Nat. Commun. 6:5164 doi: 10.1038/ncomms6164 (2014).